SLAP displays tumour suppressor functions in colorectal cancer via destabilization of the SRC substrate EPHA2 The adaptor SLAP is a negative regulator of receptor signalling in immune cells but its role in human cancer is ill defined. Here we report that SLAP is abundantly expressed in healthy epithelial intestine but strongly downregulated in 50% of colorectal cancer. SLAP overexpression suppresses cell tumorigenicity and invasiveness while SLAP silencing enhances these transforming properties. Mechanistically, SLAP controls SRC/EPHA2/AKT signalling via destabilization of the SRC substrate and receptor tyrosine kinase EPHA2. This activity is independent from CBL but requires SLAP SH3 interaction with the ubiquitination factor UBE4A and SLAP SH2 interaction with pTyr594-EPHA2. SRC phosphorylates EPHA2 on Tyr594, thus creating a feedback loop that promotes EPHA2 destruction and thereby self-regulates its transforming potential. SLAP silencing enhances SRC oncogenicity and sensitizes colorectal tumour cells to SRC inhibitors. Collectively, these data establish a tumour-suppressive role for SLAP in colorectal cancer and a mechanism of SRC oncogenic induction through stabilization of its cognate substrates. Colorectal cancer (CRC) is one of the leading causes of malignancy-related death worldwide. Most of these cancers are sporadic and under the control of genetic, epigenetic and environmental factors. When detected at early stages, CRC is curable and exhibits a 5-year survival rate of >90%. This rate decreases by ~25% at later-stage diagnosis, that is, when lymph-node metastasis is detected [1] , and occurrence of metastases in distant organs is the major cause of death for CRC patients, with a 5-year survival rate of <5% (ref. 2 ). Signalling pathways promoting metastatic progression are subject to intense investigation and tyrosine kinases (TK) have emerged as important determinants of this malignant process [3] . The non-receptor TK SRC is localized at the inner surface of the plasma membrane through N-terminal myristoylation and includes a unique N terminus, followed by SH3 and SH2 motifs, a kinase domain and a short C-terminal regulatory tail [4] . SRC coordinates intracellular signalling induced by growth factors and extracellular matrix components, leading to cell growth and adhesion. When catalytically deregulated, SRC shows oncogenic activity in rodent fibroblasts, as was originally reported for v-SRC, with a strong capacity to promote tumour growth and metastasis in experimental mouse models [4] . In human CRC, although SRC-activating mutations are rare, SRC is frequently deregulated to a level consistent with oncogenic activity [5] . Furthermore, SRC upregulation has been associated with poor clinical prognosis, suggesting an important function of SRC during metastatic progression [5] , [6] . How SRC acquires oncogenic properties in CRC cells is not clearly established. SRC deregulation primarily involves protein overexpression but it also implicates the inactivation of CSK, its major negative regulator [7] , [8] . This cytosolic TK phosphorylates SRC on Tyr529 when recruited to the plasma membrane, thus locking the enzyme in an inactive conformation. While CSK is well expressed in CRC and shows strong activity in vitro , CSK mislocalization due to the silencing of its transmembrane interactor Cbp/PAG promotes CSK inactivation and induces SRC pro-invasive activity. The nature of SRC signalling mediating this invasive process is still only partially elucidated, probably because of the capacity of SRC to phosphorylate several hundred substrates, several of them having no clear function in neoplastic transformation [9] , [10] , [11] , [12] . Interestingly, a quantitative phosphoproteomic analysis in metastatic CRC cells revealed that SRC phosphorylates a cluster of downstream TK composed of EPHA2, MET, FAK and SGK223, which were essential for the promotion of tumour cell growth and invasion [11] . EPHA2 is a Receptor Tyrosine Kinase (RTK) that binds to membrane-bound ligands called Ephrins and regulates cell–cell contacts through bidirectional signalling in neighboring cells, particularly during developmental and physiological processes [13] . Deregulation of the EPHA2/Ephrin system is frequently observed in human cancer including CRC and might participate in malignancy progression [14] . However, the exact role of EPHA2 in CRC cell tumorigenicity and invasiveness is largely unknown. Src-like adaptor protein (SLAP) belongs to the subfamily of haematopoietic adaptors that inhibit intracellular signalling. It has a unique myristoylated N terminus, followed by SH3 and SH2 domains with high homology to SRC family tyrosine kinases (SFK), and a unique C terminus with binding affinity to CBL [15] . SLAP was implicated in the negative regulation of RTK [16] , [17] and T-cell receptor (TCR) signalling [18] , [19] . Owing to its homology with the SRC-SH2 domain, SLAP competes with SRC for growth factor receptor interaction and mitogenic signalling [16] while it inhibits TCR activity by docking CBL to components of the TCR complex and inducing their degradation [20] . This mechanism may require LCK-dependent phosphorylation and the SLAP SH2 domain [20] . The SH3 domain of SLAP must also be intact for optimal attenuation of TCR signalling [19] but the nature of SH3-binders involved in this process is currently unknown. SLAP function is thought to be restricted to immune cells due to its abundance in lymphocytes [21] and the main immune defects observed in SLAP deficient mice [22] , [23] , [24] . These in vivo analyses supported a model in which SLAP dampens immunoreceptor signalling, thereby influencing lymphocyte development [15] . However, little is known about its function in other tissues or even in human cancer. SLAP has been reported to interfere with EpoR signalling in avian FLI-1-transformed erythroblasts [25] but whether SLAP has a similar role in human leukemiogenesis is currently unknown. Here we show that SLAP displays tumour suppressor function in CRC implicating the destruction of EPHA2, a key substrate for SRC function on cell tumorigenicity and invasiveness. SLAP expression appears to control the SRC oncogenic potential and CRC cell response to SRC inhibitors. Taken together, these findings reveal an important mechanism of SRC oncogenic induction in CRC and provide a rationale to predict tumour-cell response to SRC inhibitors. SLAP has a tumour-suppressive role in CRC First, we investigated whether SLAP was expressed in non-immune cells and found elevated mRNA levels in non-transformed colon epithelial cells ( Fig. 1a ). We also detected SLAP protein in macroscopically normal colon epithelium ( Fig. 1b ), whereas its expression was frequently strongly downregulated in matching CRC samples from the same patients ( Fig. 1b,c , Supplementary Fig. 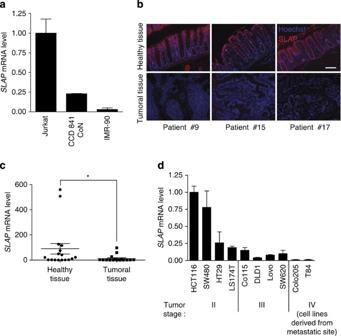Figure 1: SLAP is abundantly expressed in colon epithelium but strongly downregulated in CRC. (a)SLAmRNA level in cell lines derived from human lymphocytes (Jurkat), colonic epithelium (CCD 841 CoN) and lung (IMR-90) (means±s.e.m.;n=3). (b) Representative overlay immunofluorescence images of tumour samples and adjacent healthy tissue from three patients with CRC that were stained with Hoechst (blue) and anti-SLAP antibody (red). Scale bar, 150 μm. (c)SLAmRNA level in microdissected tumours and in adjacent healthy tissues from 17 patients with CRC (means±s.e.m.;n=17; *P<0.05, Mann–Whitney test). (d)SLAmRNA level in CRC cell lines classified according to the tumour stage (stage II–IV) (means±s.e.m.;n=3). 1 and Supplementary Table 1 ). Moreover, SLA mRNA level in CRC cell lines was inversely correlated with tumour stage ( Fig. 1d ). These data suggest that SLAP may have a role in human CRC. We thus investigated this issue further by manipulating SLAP expression in CRC cells. SLAP overexpression reduced standard proliferation of HT29 cells and anchorage-independent growth of HT29 and SW620 cells as indicated by the reduced number and size of colonies ( Fig. 2a,b and Supplementary Fig. 2a ). Similarly, growth of SLAP-overexpressing HT29 and SW620 cell xenografts was reduced ( Fig. 2c ). Conversely, shRNA-mediated SLA silencing in the HCT116 cell line, which expresses endogenous SLAP, enhanced proliferation and anchorage-independent growth in vitro as well as tumorigenicity in nude mice ( Fig. 2a–c and Supplementary Fig. 2a ). SLAP anti-oncogenic activity was next analysed in Apc Δ14/+ transgenic mice that carry a heterozygous mutation of the Apc tumour-suppressor gene and consequently develop WNT pathway-driven intestinal tumours [26] . Inhibition of SLAP expression via chronic injection of lipid-encapsulated specific siRNAs increased the number and size of tumours compared with Apc Δ14/+ mice injected with control siRNAs ( Fig. 2d–f ; see also Supplementary Fig. 3 for siRNA efficiency in cells). This finding is consistent with an essential role of SLAP downregulation in the initiation and growth of intestinal tumours that display elevated WNT pathway activity. Finally, we also observed a strong effect of SLAP on the metastatic potential of CRC cell lines. SLAP expression reduced cell migration and invasiveness, while its silencing increased them ( Fig. 2g and Supplementary Fig. 2b ). Accordingly, liver metastasis formation following intra-splenic injection of CRC HCT116 cells in nude mice was dramatically enhanced upon SLA depletion ( Fig. 2h ). We conclude that SLAP displays robust tumour suppressor functions in CRC. Figure 1: SLAP is abundantly expressed in colon epithelium but strongly downregulated in CRC. ( a ) SLA mRNA level in cell lines derived from human lymphocytes (Jurkat), colonic epithelium (CCD 841 CoN) and lung (IMR-90) (means±s.e.m. ; n =3). ( b ) Representative overlay immunofluorescence images of tumour samples and adjacent healthy tissue from three patients with CRC that were stained with Hoechst (blue) and anti-SLAP antibody (red). Scale bar, 150 μm. ( c ) SLA mRNA level in microdissected tumours and in adjacent healthy tissues from 17 patients with CRC (means±s.e.m. ; n =17; * P <0.05, Mann–Whitney test). ( d ) SLA mRNA level in CRC cell lines classified according to the tumour stage (stage II–IV) (means±s.e.m. ; n =3). 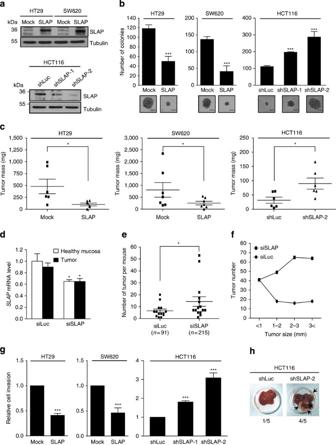Figure 2: SLAP controls CRC cell tumorigenicity and invasiveness. (a) HT29 and SW620 cells were infected with retroviral vectors that express SLAP (top). HCT116 cells were infected with retroviral vectors that express shRNAs targetingSLA(shSLAP) or Luciferase (shLuc) as control (bottom). SLAP protein level was analysed by immunoblotting. Tubulin was used as loading control. (b) SLAP affects anchorage-independent growth. Number of colonies obtained from cells infected with the indicated vectors and grown in soft agar (top) (means±s.e.m.;n=4; ***P<0.001, Student’sttest). Representative images of the colonies (bottom). Scale bar, 200 μm. (c) SLAP affects subcutaneous tumour growth. Cells infected with the indicated vectors were inoculated s.c. in nude mice. Graphs show the mass of the isolated tumours at day 35 post-graft (means±s.e.m.;n=6–7 mice/group; *P<0.05, Student’sttest). (d–f) SLAP depletion increases the number and size of intestinal tumours inAPCΔ14/+mice.APCΔ14/+mice were treated with siRNAs targeting Luciferase (siLuc) orSlap(siSLAP) by using the siSLAPm2 sequence tested inSupplementary Fig. 3. (d)SlapmRNA level in adenomas and adjacent healthy mucosa (means±s.e.m.;n=32 for siLuc-treated mice andn=56 for siSLAP-treated mice; *P<0.05 Student’st-test). (e) Number of tumours per mouse (means±s.e.m.;n=15 mice per group; *P<0.05, Mann–Whitney test). The total number of tumours per group is indicated underneath. (f) Number of tumours for each size group. (g) SLAP hinders CRC cell invasion in Boyden chamber assays. Invasion of CRC cells infected with the indicated vectors was expressed relative to the control (mock or shLuc) value that was arbitrarily set at 1 (means±s.e.m.;n=6; ***P<0.001 Student’st-test). (h)SLAdepletion in HCT116 cells promotes liver metastasis formation. HCT116 cells infected with the indicated vectors were inoculated in the spleen of nude mice. After 2 weeks, livers were removed. A representative liver image is shown for each group. Arrows show the liver nodules. The number of mice with nodules is indicated for each group. Full size image Figure 2: SLAP controls CRC cell tumorigenicity and invasiveness. ( a ) HT29 and SW620 cells were infected with retroviral vectors that express SLAP (top). HCT116 cells were infected with retroviral vectors that express shRNAs targeting SLA (shSLAP) or Luciferase (shLuc) as control (bottom). SLAP protein level was analysed by immunoblotting. Tubulin was used as loading control. ( b ) SLAP affects anchorage-independent growth. Number of colonies obtained from cells infected with the indicated vectors and grown in soft agar (top) (means±s.e.m. ; n =4; *** P <0.001, Student’s t test). Representative images of the colonies (bottom). Scale bar, 200 μm. ( c ) SLAP affects subcutaneous tumour growth. Cells infected with the indicated vectors were inoculated s.c. in nude mice. Graphs show the mass of the isolated tumours at day 35 post-graft (means±s.e.m. ; n =6–7 mice/group; * P <0.05, Student’s t test). ( d – f ) SLAP depletion increases the number and size of intestinal tumours in APC Δ14/+ mice. APC Δ14/+ mice were treated with siRNAs targeting Luciferase (siLuc) or Slap (siSLAP) by using the siSLAPm2 sequence tested in Supplementary Fig. 3 . ( d ) Slap mRNA level in adenomas and adjacent healthy mucosa (means±s.e.m. ; n =32 for siLuc-treated mice and n =56 for siSLAP-treated mice; * P <0.05 Student’s t -test). ( e ) Number of tumours per mouse (means±s.e.m. ; n =15 mice per group; * P <0.05, Mann–Whitney test). The total number of tumours per group is indicated underneath. ( f ) Number of tumours for each size group. ( g ) SLAP hinders CRC cell invasion in Boyden chamber assays. Invasion of CRC cells infected with the indicated vectors was expressed relative to the control (mock or shLuc) value that was arbitrarily set at 1 (means±s.e.m. ; n =6; *** P <0.001 Student’s t -test). ( h ) SLA depletion in HCT116 cells promotes liver metastasis formation. HCT116 cells infected with the indicated vectors were inoculated in the spleen of nude mice. After 2 weeks, livers were removed. A representative liver image is shown for each group. Arrows show the liver nodules. The number of mice with nodules is indicated for each group. Full size image SLAP controls SRC oncogenic signalling via destabilization of EPHA2 The molecular mechanism by which SLAP inhibits oncogenic signalling was next addressed. The control of cell transformation by SLAP was dependent on SFK activity as SFK inhibition abrogated the enhancement of soft agar colony formation and invasiveness due to SLAP silencing ( Fig. 3a ). Conversely, SLAP antagonized SRC cell transforming activity in HT29 and SW620 cells ( Fig. 3b,c ). However, SLAP did not alter SRC activity (pY418), SRC-induced FAK activity (pY861) and Tyr phosphorylation (pTyr), suggesting that this adaptor targets a downstream component of SRC signalling ( Fig. 3c,d ). To further investigate the mechanism underlying SLAP tumour suppressor role, we used SLAP mutants that harbour a mutation in the SH2 and/or SH3 domains (SH2*, SH3*, SH3*SH2*) or in the myristylated site (G2A), or a deletion of the C-terminal domain (N32). This structure–function analysis revealed that the SH2 and SH3 domains as well as membrane localization were required for SLAP inhibitory function, whereas the C terminus was dispensable, thus excluding a CBL-dependent mechanism ( Fig. 4a–c ). Moreover, although SLAP expression did not significantly affect the global pTyr level in these cells, it modulated the pTyr level of and co-immunoprecipitated with a 130-kDa protein in a SH2 and SH3 domain-dependent manner ( Fig. 4d,e ). The identity of this protein was unravelled via a SILAC-based quantitative proteomic analysis, which allowed the identification of SLAP interactors in tumour cells including those phosphorylated on tyrosine residues. A prominent interactor isolated was EPHA2, which we recently described as an important SRC substrate for oncogenic signalling [11] . While SLAP was originally identified by its binding capacity to EPHA2, their interaction has never been addressed in vivo [21] . We confirmed the existence of SLAP–EPHA2 complexes in CRC cells ( Fig. 4f ) and demonstrated the requirement of intact SLAP SH2 and -SH3 domains for this interaction ( Fig. 4g and Supplementary Fig. 4 ). Furthermore, in agreement with the previously reported detection of Tyr594-phosphorylated EPHA2 in cancer cells ( www.phosphosite.org ) and with its predicted high affinity for SLAP SH2 (ref. 27 ), the use of an EPHA2 variant with a mutation in Tyr594 demonstrated that Tyr594 is essential for SLAP binding to EPHA2 ( Fig. 4h ). 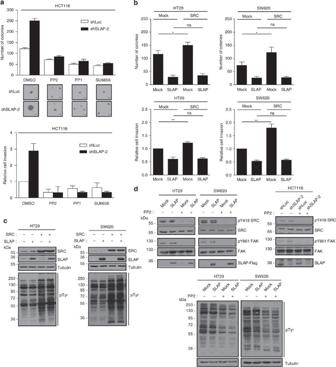Figure 3: SLAP antagonizes SRC oncogenic signalling. (a) SRC inhibition reverses the transforming properties induced by SLAP depletion in CRC cells. HCT116 cells that express anti-SLAP(shSLAP) or anti-Luciferase (shLuc) shRNAs were treated with the SRC inhibitors PP2 (5 μM), PP1 (5 μM), SU6656 (5 μM) or vehicle (DMSO). Left panel: quantification of the colonies obtained from cells that express the indicated shRNAs and were grown in soft agar (top). Representative images of the obtained colonies (bottom). Scale bar, 200 μm. Right panel: Boyden chamber assays; histograms show the invasion of cells that express the indicated shRNAs relative to control (HCT116-shLuc cells treated with DMSO), arbitrarily set at 1. Data represent means±s.e.m.;n=4. (b,c) SRC overexpression does not rescue the transforming properties inhibited by SLAP in CRC cells. HT29 and SW620 cells were infected with the indicated viruses. (b) Upper panel: soft agar colony formation assay. Lower panel: invasion assay. Data represent means±s.e.m.;n=5; ns, not significant, *P<0.05, **P<0.01 (Student’sttest). (c) Cell lysates were analysed by immunoblotting. (d) SLAP does not inhibit SRC activity. HT29, SW620 and HCT116 cells infected with the indicated viruses were treated with the SRC inhibitor PP2 (5 μM) or vehicle (DMSO) for 4 h. Cell lysates were analyzed by immunoblotting. Figure 3: SLAP antagonizes SRC oncogenic signalling. ( a ) SRC inhibition reverses the transforming properties induced by SLAP depletion in CRC cells. HCT116 cells that express anti- SLAP (shSLAP) or anti-Luciferase (shLuc) shRNAs were treated with the SRC inhibitors PP2 (5 μM), PP1 (5 μM), SU6656 (5 μM) or vehicle (DMSO). Left panel: quantification of the colonies obtained from cells that express the indicated shRNAs and were grown in soft agar (top). Representative images of the obtained colonies (bottom). Scale bar, 200 μm. Right panel: Boyden chamber assays; histograms show the invasion of cells that express the indicated shRNAs relative to control (HCT116-shLuc cells treated with DMSO), arbitrarily set at 1. Data represent means±s.e.m. ; n =4. ( b , c ) SRC overexpression does not rescue the transforming properties inhibited by SLAP in CRC cells. HT29 and SW620 cells were infected with the indicated viruses. ( b ) Upper panel: soft agar colony formation assay. Lower panel: invasion assay. Data represent means±s.e.m. ; n =5; ns, not significant, * P <0.05, ** P <0.01 (Student’s t test). ( c ) Cell lysates were analysed by immunoblotting. ( d ) SLAP does not inhibit SRC activity. HT29, SW620 and HCT116 cells infected with the indicated viruses were treated with the SRC inhibitor PP2 (5 μM) or vehicle (DMSO) for 4 h. Cell lysates were analyzed by immunoblotting. 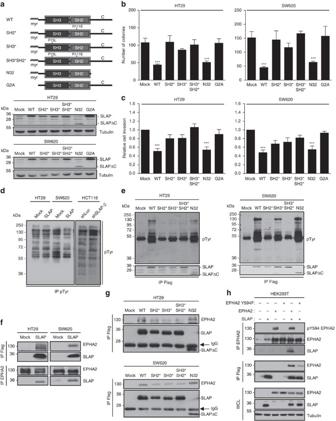Figure 4: SLAP interacts with EPHA2 in CRC cells. (a–c) SLAP function requires intact SH2 and SH3 domains as well as membrane localization. (a) HT29 and SW620 cells were infected with retroviral vectors expressing the indicated SLAP mutants. Upper panel: schematic representation of the SLAP mutants used in this study. Myristyl group (myr), C-terminal domain (C) and SH3 or SH2 point mutations are indicated. Lower panel: SLAP protein level in the indicated cell lysates was analysed by immunoblotting. (b) Soft agar colony formation assay and (c) Invasion assay. Data in (b) and (c) represent means±s.e.m.;n=6; ***P<0.001 (Student’st-test). (d) SLAP weakly affects the global level of pTyr in CRC cells. pTyr proteins from CRC cell lines infected with the indicated vectors were immunoprecipitated (IP) and immunoblotted (IB) with the 4G10 antibody. (e) SLAP interacts with pTyr proteins in CRC cells. SLAP-Flag proteins from the indicated cell lysates were immunoprecipitated with anti-Flag M2 agarose affinity gel. pTyr proteins interacting with SLAP were detected by IB with the 4G10 antibody. The levels of immunoprecipitated SLAP are also shown. (f) SLAP interacts with EPHA2 in CRC cells. The levels of SLAP-Flag and EPHA2 co-IP by the indicated antibodies from cell lysates were analysed by IB. (g) The interaction between SLAP and EPHA2 requires intact SH2 and SH3 domains. The levels of SLAP-Flag and EPHA2 co-IP by the anti-Flag antibody from cell lysates were analysed by IB. (h) The interaction between SLAP and EPHA2 requires phosphorylation of EPHA2 at Tyr594. HEK293T cells were transfected with the indicated constructs for 48 h. Cell lysates were IP with the indicated antibodies. Whole cell lysates (WCL) and immunoprecipitates were analyzed by IB. Full size image Figure 4: SLAP interacts with EPHA2 in CRC cells. ( a – c ) SLAP function requires intact SH2 and SH3 domains as well as membrane localization. ( a ) HT29 and SW620 cells were infected with retroviral vectors expressing the indicated SLAP mutants. Upper panel: schematic representation of the SLAP mutants used in this study. Myristyl group (myr), C-terminal domain (C) and SH3 or SH2 point mutations are indicated. Lower panel: SLAP protein level in the indicated cell lysates was analysed by immunoblotting. ( b ) Soft agar colony formation assay and ( c ) Invasion assay. Data in ( b ) and ( c ) represent means±s.e.m. ; n =6; *** P <0.001 (Student’s t -test). ( d ) SLAP weakly affects the global level of pTyr in CRC cells. pTyr proteins from CRC cell lines infected with the indicated vectors were immunoprecipitated (IP) and immunoblotted (IB) with the 4G10 antibody. ( e ) SLAP interacts with pTyr proteins in CRC cells. SLAP-Flag proteins from the indicated cell lysates were immunoprecipitated with anti-Flag M2 agarose affinity gel. pTyr proteins interacting with SLAP were detected by IB with the 4G10 antibody. The levels of immunoprecipitated SLAP are also shown. ( f ) SLAP interacts with EPHA2 in CRC cells. The levels of SLAP-Flag and EPHA2 co-IP by the indicated antibodies from cell lysates were analysed by IB. ( g ) The interaction between SLAP and EPHA2 requires intact SH2 and SH3 domains. The levels of SLAP-Flag and EPHA2 co-IP by the anti-Flag antibody from cell lysates were analysed by IB. ( h ) The interaction between SLAP and EPHA2 requires phosphorylation of EPHA2 at Tyr594. HEK293T cells were transfected with the indicated constructs for 48 h. Cell lysates were IP with the indicated antibodies. Whole cell lysates (WCL) and immunoprecipitates were analyzed by IB. Full size image We next investigated the effect of SLAP interaction on EPHA2 activity. In CRC cell lines, SLAP tightly controlled EPHA2 protein expression but not its transcript level ( Fig. 5a and Supplementary Fig. 5a ). Similarly, in CRC samples ( Fig. 5b and Supplementary Fig. 5b,c ) and experimental tumour models ( Supplementary Fig. 5d ), the abundance of EPHA2 protein was inversely correlated with SLAP expression, while the level of EPHA2 transcript was not modified. The decrease of cellular EPHA2 in the presence of SLAP was specifically reversed by treatment with the proteasome inhibitor MG132 ( Fig. 5c and Supplementary Fig. 6 ), implicating a proteasome-dependent mechanism in EPHA2 destabilization. Furthermore, the capacity of SLAP to regulate EPHA2 protein stability required the SH2 and SH3 domains, which are also needed for its anti-oncogenic functions ( Fig. 5d ). To investigate whether EPHA2 destabilization is essential for SLAP anti-oncogenic role, EPHA2 protein level in SLAP-expressing cells was restored by using a retroviral EPHA2 construct. While forced expression of EPHA2 had a moderate effect on the transforming properties of control cells, it strongly antagonized the robust anti-oncogenic effect of SLAP ( Fig. 5e ). Likewise, EPHA2 silencing reversed the increased transforming properties induced by SLA silencing in HCT116 cells, while it did not have any major effect in control cells ( Fig. 5f ). Overall, these data corroborate the hypothesis that SLAP anti-oncogenic activity is mediated by proteasomal degradation of EPHA2. 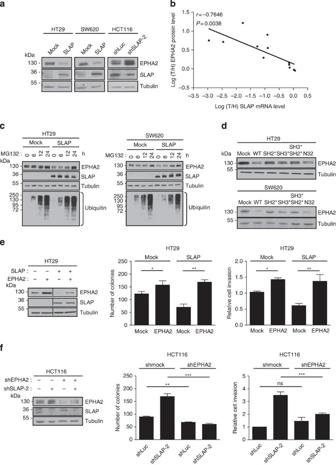Figure 5: SLAP anti-oncogenic activity is mediated by proteasomal degradation of EPHA2. (a) SLAP decreases EPHA2 protein levels in CRC cells. Immunoblot (IB) analysis showing the levels of SLAP, EPHA2 and Tubulin in the lysates from CRC cell lines infected with the indicated vectors. (b) Inverse correlation betweenSLAmRNA level and EPHA2 protein level in CRC samples.SLAmRNA level was measured by qPCR in microdissected tumours (T) and in the adjacent healthy tissue (H) from 12 patients with CRC. EPHA2 protein level was analysed in tumour (T) and adjacent healthy tissue (H) samples from the same patients by IB. Signal intensities were quantified using the Image J software.r, Pearson correlation’s coefficient. (c) SLAP induces EPHA2 proteasomal degradation. HT29 and SW620 cells infected with the indicated vectors were treated with the proteasome inhibitor MG132 (5 μM) or vehicle (DMSO; dimethyl sulfoxide) for the indicated times. The levels of SLAP, EPHA2, Tubulin and ubiquitinated proteins in lysates were analysed by IB. (d) SLAP-dependent EPHA2 degradation requires intact SH2 and SH3 domains. The levels of EPHA2 and Tubulin from lysates of cells that express the indicated SLAP mutants were analysed by IB. (e) EPHA2 expression antagonizes SLAP function. HT29 cells were infected with the indicated viruses. Left panel: IB analysis. Vertical black lines denote that lanes were non-adjacent in the gel. Middle panel: soft agar colony formation assay. Right panel: invasion assay. Data represent means±s.e.m.;n=3; *P<0.05, **P<0.01 (Student’st-test). (f) EPHA2 depletion reverses the transforming properties induced by SLAP inactivation. HCT116 cells were infected with the indicated viruses. Left panel: IB analysis. Middle panel: soft agar colony formation assay. Right panel: invasion assay. Data represent means±s.e.m.;n=5; ns, not significant, **P<0.01, ***P<0.001 (Student’st-test). Figure 5: SLAP anti-oncogenic activity is mediated by proteasomal degradation of EPHA2. ( a ) SLAP decreases EPHA2 protein levels in CRC cells. Immunoblot (IB) analysis showing the levels of SLAP, EPHA2 and Tubulin in the lysates from CRC cell lines infected with the indicated vectors. ( b ) Inverse correlation between SLA mRNA level and EPHA2 protein level in CRC samples. SLA mRNA level was measured by qPCR in microdissected tumours (T) and in the adjacent healthy tissue (H) from 12 patients with CRC. EPHA2 protein level was analysed in tumour (T) and adjacent healthy tissue (H) samples from the same patients by IB. Signal intensities were quantified using the Image J software. r , Pearson correlation’s coefficient. ( c ) SLAP induces EPHA2 proteasomal degradation. HT29 and SW620 cells infected with the indicated vectors were treated with the proteasome inhibitor MG132 (5 μM) or vehicle (DMSO; dimethyl sulfoxide) for the indicated times. The levels of SLAP, EPHA2, Tubulin and ubiquitinated proteins in lysates were analysed by IB. ( d ) SLAP-dependent EPHA2 degradation requires intact SH2 and SH3 domains. The levels of EPHA2 and Tubulin from lysates of cells that express the indicated SLAP mutants were analysed by IB. ( e ) EPHA2 expression antagonizes SLAP function. HT29 cells were infected with the indicated viruses. Left panel: IB analysis. Vertical black lines denote that lanes were non-adjacent in the gel. Middle panel: soft agar colony formation assay. Right panel: invasion assay. Data represent means±s.e.m. ; n =3; * P <0.05, ** P <0.01 (Student’s t -test). ( f ) EPHA2 depletion reverses the transforming properties induced by SLAP inactivation. HCT116 cells were infected with the indicated viruses. Left panel: IB analysis. Middle panel: soft agar colony formation assay. Right panel: invasion assay. Data represent means±s.e.m. ; n =5; ns, not significant, ** P <0.01, *** P <0.001 (Student’s t -test). Full size image UBE4A mediates SLAP-induced EPHA2 degradation We then investigated the mechanism by which SLAP promotes EPHA2 destabilization. In contrast to previous reports [15] , [17] , [20] , CBL was not involved in this process. Specifically, CBL did not interact with SLAP in CRC cell lines ( Supplementary Fig. 7a ) and SLAP activity was not affected by the deletion of its CBL-binding domain or by CBL silencing ( Fig. 4b,c and Supplementary Fig. 7b ). UBE3C and LTN1, two additional E3 ligases identified in our proteomic analysis ( www.peptideatlas.org/PASS/PASS00376 ), were not involved either ( Supplementary Fig. 7c,d ). In contrast, UBE4A, the human homologue of the yeast UFD2 ubiquitination factor [28] , was a major SLAP interactor in CRC cells. Indeed, SLAP co-precipitated with UBE4A in CRC cells and their association also required the SH3 domain of SLAP ( Fig. 6a,b ). This result was confirmed by GST pull-down assays using purified proteins, indicating that UBE4A binds directly to the SLAP SH3 domain ( Fig. 6c ). In addition, UBE4A co-precipitated with EPHA2 in a SLAP-dependent manner, probably due to the capacity of SLAP to form dimers and therefore to interact with two SH3-binding molecules [29] ( Fig. 6d ). We next assessed the capacity of UBE4A to promote EPHA2 ubiquitination. While SLAP or UBE4A alone had no clear effect, co-expressed molecules dramatically increased EPHA2 ubiquitination in HEK293 cells ( Fig. 6e ). This effect required the SLAP SH3 and SH2 domains as well as a functional UBE4A-U box that harbours Ubiquitin ligase activity [28] ( Fig. 6f ). Purified UBE4A also ubiquitinated EPHA2 in vitro , demonstrating that EPHA2 is a direct substrate of UBE4A ( Fig. 6g ). These results are consistent with a model in which SLAP mediates EPHA2–UBE4A interaction and thereby promotes proteasomal degradation of EPHA2. Accordingly, the capacity of SLAP to reduce EPHA2 protein abundance was attenuated by UBE4A silencing in HT29 cells ( Fig. 6h ). A partial effect was observed in SW620 cells, suggesting the existence of an additional mechanism in these cells ( Supplementary Fig. 7e ). Finally, SLAP anti-oncogenic effects were compromised by UBE4A depletion ( Fig. 6i and Supplementary Fig. 7e ). We thus conclude that UBE4A is an essential mediator of SLAP anti-oncogenic activity in tumour cells. 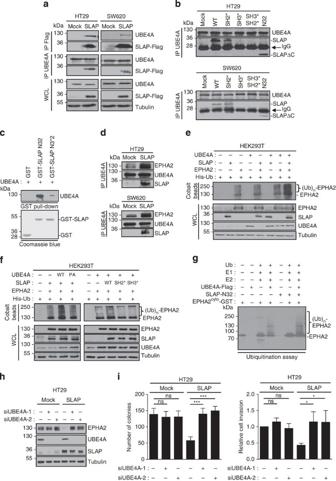Figure 6: UBE4A mediates SLAP anti-oncogenic activity. (a) SLAP interacts with UBE4A in CRC cells. The levels of SLAP and UBE4A in whole-cell lysates (WCL) and in samples co-immunoprecipitated (IP) by the indicated antibodies were analysed by immunoblotting (IB). (b) The interaction between SLAP and UBE4A requires an intact SH3 domain. The levels of SLAP and UBE4A co-IP with an anti-UBE4A antibody from lysates of cells that express the indicated SLAP mutants were analysed by IB. (c) Direct interaction between SLAP and UBE4A by GST pull-down assays. Indicated GST-fusion proteins and UBE4A were mixed. The levels of UBE4A precipitated with Gluthatione beads were analysed by IB. Coomassie blue staining shows the level of precipitated fusion proteins. (d) The interaction between EPHA2 and UBE4A in CRC cells is SLAP-dependent. The levels of SLAP, UBE4A and EPHA2 co-IP by an anti-UBE4A antibody from the indicated cell lysates were analysed by IB. (e) EPHA2 ubiquitination is induced by the SLAP–UBE4A complex. HEK293T cells were transfected with the indicated constructs and His-tagged ubiquitin (Ub-His). After 48 h, cells were treated with 10 μM MG132 for 4 h and lysed in denaturing conditions. Ubiquitinated proteins were purified using cobalt beads. WCL and precipitates were analysed by IB. (f) EPHA2 ubiquitination induced by the SLAP–UBE4A complex requires the SH3 and SH2 SLAP domains and a functional UBE4A-U box domain. HEK293T cells were transfected for 2 d with SLAP, EPHA2 and Histidine-tagged Ubiquitin (His-Ub) constructs as indicated, in the presence or absence of wild type (WT) or catalytically inactive UBE4A/P1030A mutant (PA), as shown, treated with 10 μM MG132 for 4 h and lysed in denaturing conditions. Ubiquitinated proteins were purified using cobalt beads. WCL and precipitates were analysed by IB. (g) UBE4A mediates EPHA2 ubiquitinationin vitro. Ubiquitination assays were performed with the indicated proteins in the presence of Ubiquitin (Ub), E1 and UbcH5B (E2) and analysed by IB with an anti-EPHA2 antibody. (h) SLAP-dependent EPHA2 degradation is mediated by UBE4A. HT29 cells expressing SLAP or not were transfected with siRNAs targetingUBE4A(+) or control siRNAs (−) for 72 h. Cell lysates were analysed by IB. (i) UBE4A depletion reverses SLAP anti-oncogenic activity. Left panel: soft agar colony formation assay. Right panel: invasion assay. Data represent means±s.e.m.;n=3. ns, not significant, *P<0.05, ***P<0.001 (Student’st-test). Figure 6: UBE4A mediates SLAP anti-oncogenic activity. ( a ) SLAP interacts with UBE4A in CRC cells. The levels of SLAP and UBE4A in whole-cell lysates (WCL) and in samples co-immunoprecipitated (IP) by the indicated antibodies were analysed by immunoblotting (IB). ( b ) The interaction between SLAP and UBE4A requires an intact SH3 domain. The levels of SLAP and UBE4A co-IP with an anti-UBE4A antibody from lysates of cells that express the indicated SLAP mutants were analysed by IB. ( c ) Direct interaction between SLAP and UBE4A by GST pull-down assays. Indicated GST-fusion proteins and UBE4A were mixed. The levels of UBE4A precipitated with Gluthatione beads were analysed by IB. Coomassie blue staining shows the level of precipitated fusion proteins. ( d ) The interaction between EPHA2 and UBE4A in CRC cells is SLAP-dependent. The levels of SLAP, UBE4A and EPHA2 co-IP by an anti-UBE4A antibody from the indicated cell lysates were analysed by IB. ( e ) EPHA2 ubiquitination is induced by the SLAP–UBE4A complex. HEK293T cells were transfected with the indicated constructs and His-tagged ubiquitin (Ub-His). After 48 h, cells were treated with 10 μM MG132 for 4 h and lysed in denaturing conditions. Ubiquitinated proteins were purified using cobalt beads. WCL and precipitates were analysed by IB. ( f ) EPHA2 ubiquitination induced by the SLAP–UBE4A complex requires the SH3 and SH2 SLAP domains and a functional UBE4A-U box domain. HEK293T cells were transfected for 2 d with SLAP, EPHA2 and Histidine-tagged Ubiquitin (His-Ub) constructs as indicated, in the presence or absence of wild type (WT) or catalytically inactive UBE4A/P1030A mutant (PA), as shown, treated with 10 μM MG132 for 4 h and lysed in denaturing conditions. Ubiquitinated proteins were purified using cobalt beads. WCL and precipitates were analysed by IB. ( g ) UBE4A mediates EPHA2 ubiquitination in vitro . Ubiquitination assays were performed with the indicated proteins in the presence of Ubiquitin (Ub), E1 and UbcH5B (E2) and analysed by IB with an anti-EPHA2 antibody. ( h ) SLAP-dependent EPHA2 degradation is mediated by UBE4A. HT29 cells expressing SLAP or not were transfected with siRNAs targeting UBE4A (+) or control siRNAs (−) for 72 h. Cell lysates were analysed by IB. ( i ) UBE4A depletion reverses SLAP anti-oncogenic activity. Left panel: soft agar colony formation assay. Right panel: invasion assay. Data represent means±s.e.m. ; n =3. ns, not significant, * P <0.05, *** P <0.001 (Student’s t -test). Full size image SLAP hinders SRC/EPHA2/AKT signalling We next evaluated the nature of EPHA2 signalling targeted by SLAP in tumour cells. Ephrin binding induces rapid EPHA2 kinase activation, followed by CBL-dependent receptor degradation [30] . As SLAP defines an additional mechanism of EPHA2 destabilization, we investigated whether SLAP also plays a role in Ephrin-A1-induced EPHA2 degradation. SLAP had a strong impact on the basal level of EPHA2, but it did not affect Ephrin-A1-induced receptor activation and protein degradation ( Fig. 7a and Supplementary Fig. 8a ). Likewise, SLAP-induced EPHA2 destabilization was not modified in cells plated at low density, which prevents cell interaction and receptor activation induced by endogenous Ephrins ( Supplementary Fig. 8b ). These data are consistent with a model where SLAP induces Ephrin-independent EPHA2 degradation. It also suggests that EPHA2 has a ligand-independent function in tumour cells. Accordingly, while Ephrin-A1 induced a dramatic increase in EPHA2 activity, it did not rescue the SLAP-mediated inhibition of cell transformation ( Fig. 7a ). Furthermore, Ephrin-A1 slightly reduced cell transformation that was increased upon SLAP silencing ( Fig. 7a ). We thus conclude that SLAP targets a ligand-independent function of EPHA2. We then tried to identify the molecular determinants involved in SLAP-regulated EPHA2 signalling. As restoration of EPHA2 protein level in SLAP-expressing cells fully antagonized SLAP activity, we analysed the capacity of EPHA2 mutants to induce a similar rescuing effect. Surprisingly, the catalytically inactive kinase dead (KD)-EPHA2 mutant retained the full capacity to antagonize SLAP activity, consistent with an adaptor function of EPHA2 in tumour cells ( Fig. 7b,c and Supplementary Fig. 9a ). Moreover, although the Y594F-EPHA2 mutant was more stable because of its incapacity to interact with SLAP, it did not restore cell transformation in SLAP-expressing cells ( Fig. 7b,c and Supplementary Fig. 9a ). It is therefore likely that this phosphorylation site is included in the binding motif of an additional signalling molecule required for cell transformation. Accordingly, (KD)-EPHA2 mutant was also phosphorylated on Tyr594 and its full capacity to antagonize SLAP activity was also dependent on this residue ( Supplementary Fig. 9b,c ). It should be noted that EPHA2 rescuing effects were inhibited by a SRC inhibitor, in agreement with the existence of a SRC-EPHA2 signalling mechanism in these cells ( Supplementary Fig. 9d ). Altogether, these data uncover a novel SRC-induced and ligand-independent adaptor function of EPHA2 in CRC cells. 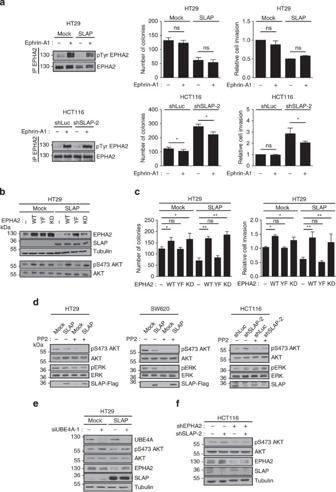Figure 7: SLAP hinders a SRC/EPHA2/AKT signalling cascade. (a) Ligand-independent function of EPHA2 in CRC cells. HT29 and HCT116 cells infected with the indicated viruses were stimulated with 1 μg ml−1pre-clustered Ephrin-A1-Fc or Fc (control). Left panel: after 15 min stimulation, cell lysates were immunoprecipitated (IP) with a limited amount of anti-EPHA2 antibody. Immunoprecipitates were analysed by immunoblotting (IB). Middle panel: Soft agar colony formation assay. Right panel: invasion assay. Data represent means±s.e.m.;n=3. ns, not significant, *P<0.05 (Student’sttest). (b,c) Adaptor function of EPHA2 in CRC cells. HT29 cells expressing SLAP or not (mock) were infected with retroviral vectors that express the indicated EPHA2 mutants (WT, wild type; YF, Y594F mutant and KD, kinase dead) (b) Cell lysates were analysed by IB. (c) Left panel: soft agar colony formation assay. Right panel: invasion assay. Data represent means±s.e.m.;n=3. ns, not significant, *P<0.05, **P<0.01 (Student’sttest). (d) SLAP controls AKT activity in CRC cells. HT29, SW620 and HCT116 cells infected with the indicated viruses were treated with the SRC inhibitor PP2 (5 μM) or vehicle (DMSO) for 4 h. Cell lysates were analysed by IB. (e)UBE4Asilencing reverses SLAP-mediated AKT inhibition. HT29 cells that express SLAP or not were transfected with siRNA targetingUBE4A(+) or siRNA negative control (−) for 72 h. Cell lysates were analyzed by IB. (f)EPHA2silencing reverses AKT activation induced by SLAP depletion. HCT116 cells were infected with the indicated viruses. Cell lysates were analysed by IB. Figure 7: SLAP hinders a SRC/EPHA2/AKT signalling cascade. ( a ) Ligand-independent function of EPHA2 in CRC cells. HT29 and HCT116 cells infected with the indicated viruses were stimulated with 1 μg ml −1 pre-clustered Ephrin-A1-Fc or Fc (control). Left panel: after 15 min stimulation, cell lysates were immunoprecipitated (IP) with a limited amount of anti-EPHA2 antibody. Immunoprecipitates were analysed by immunoblotting (IB). Middle panel: Soft agar colony formation assay. Right panel: invasion assay. Data represent means±s.e.m. ; n =3. ns, not significant, * P <0.05 (Student’s t test). ( b , c ) Adaptor function of EPHA2 in CRC cells. HT29 cells expressing SLAP or not (mock) were infected with retroviral vectors that express the indicated EPHA2 mutants (WT, wild type; YF, Y594F mutant and KD, kinase dead) ( b ) Cell lysates were analysed by IB. ( c ) Left panel: soft agar colony formation assay. Right panel: invasion assay. Data represent means±s.e.m. ; n =3. ns, not significant, * P <0.05, ** P <0.01 (Student’s t test). ( d ) SLAP controls AKT activity in CRC cells. HT29, SW620 and HCT116 cells infected with the indicated viruses were treated with the SRC inhibitor PP2 (5 μM) or vehicle (DMSO) for 4 h. Cell lysates were analysed by IB. ( e ) UBE4A silencing reverses SLAP-mediated AKT inhibition. HT29 cells that express SLAP or not were transfected with siRNA targeting UBE4A (+) or siRNA negative control (−) for 72 h. Cell lysates were analyzed by IB. ( f ) EPHA2 silencing reverses AKT activation induced by SLAP depletion. HCT116 cells were infected with the indicated viruses. Cell lysates were analysed by IB. Full size image We next started the analysis of the EPHA2-dependent intracellular signalling components affected by SLAP. SLAP did not have any effect on MAPK signalling, but reduced the Ser473 phosphorylation of AKT ( Fig. 7d ). AKT activity was also strongly reduced by PP2, an SFK inhibitor, suggesting that this signalling pathway is under the control of SFK activity ( Fig. 7d ). Moreover, an AKT inhibitor reversed the increase in transforming properties induced by SLA silencing, thus revealing an important role of AKT in SLAP anti-oncogenic activity ( Supplementary Fig. 10 ). As EPHA2 is targeted by the SLAP–UBE4A complex, we hypothesized that SLAP effect on AKT largely relies on EPHA2 destabilization. Indeed, SLAP-induced AKT inhibition was fully dependent on the expression of UBE4A and EPHA2 ( Fig. 7e,f ). Moreover, expression of wild type or KD-EPHA2 fully reversed the SLAP inhibitory effect on AKT activity ( Fig. 7b ). In contrast, both Y594F-EPHA2 and Y594F-(KD)-EPHA2, which failed to restore cell transformation, did not rescue AKT activity either ( Fig. 7b and Supplementary Fig. 9c ). This finding suggests that phosphorylation of EPHA2 on Tyr594 mediates AKT activation. We thus conclude that SLAP hinders a SRC/EPHA2/AKT signalling cascade in CRC cells. SRC regulates SLAP anti-oncogenic activity Our data show that SLAP signalling is controlled by phosphorylation of EPHA2 on Tyr594. As EPHA2 is a SRC substrate, we hypothesized that SRC itself could promote SLAP signalling by phosphorylating this residue. Indeed SRC phosphorylates EPHA2 on Tyr594 both in vitro and in vivo ( Fig. 8a–c and Supplementary Fig. 11a ). SRC also associated with EPHA2, but pTyr594 was not involved in this interaction, differently from what was observed for SLAP ( Supplementary Fig. 11b ). Accordingly, SLAP overexpression did not affect SRC–EPHA2 complex formation ( Supplementary Fig. 11c ). Therefore, SLAP may not compete with SRC for EPHA2 interaction, unlike for other RTKs [16] , [17] . Moreover SRC silencing or inhibition reduced the association of SLAP with EPHA2 ( Fig. 8a,b and Supplementary Fig. 11a ). Consequently, the EPHA2 protein level was increased upon acute SRC inhibition in CRC cells, an effect that was fully dependent on SLAP expression ( Fig. 8d,e ). Also, SRC expression increased EPHA2 degradation in SW620 tumour cells, which retain a residual level of EPHA2 following SLAP expression ( Fig. 8f ) and in HCT116 cells, which express endogenous SLAP ( Fig. 8g ). Conversely, SRC-induced EPHA2 destabilization was abrogated by SLA silencing ( Fig. 8g ). We therefore conclude that SRC initiates a regulatory loop through the promotion of SLAP–EPHA2 complex formation, leading to EPHA2 degradation. 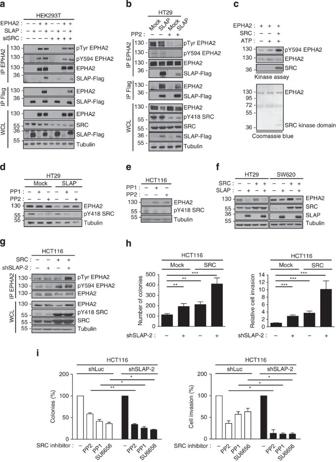Figure 8: SLAP controls the SRC oncogenic potential and the cell response to SRC inhibitors. (a,b) The interaction between SLAP and EPHA2 is SRC-dependent. (a) HEK293T were transfected with the indicated constructs and with siRNA targetingSRC(+) or siRNA negative control (−). 72 h after transfection, cell lysates were immunoprecipitated (IP) with the indicated antibodies. Whole-cell lysates (WCL) and immunoprecipitates were analysed by immunoblotting (IB). (b) HT29 cells expressing SLAP or not were treated with the SRC inhibitor PP2 (5 μM) or vehicle (DMSO) for 4 h. Cell lysates were IP with the indicated antibodies. WCL and immunoprecipitates were analysed by IB. (c) SRC phosphorylates EPHA2in vitro. Indicated proteins were incubated with or without ATP. The levels of pY594-EPHA2, EPHA2 and SRC were analysed by IB. (d–f) SRC mediates SLAP-dependent EPHA2 destabilization. HT29 cells that express SLAP or not (d) and HCT116 cells (e) were treated with the SRC inhibitors PP1 (5 μM), PP2 (5 μM) or vehicle (DMSO) for 4 h. Cell lysates were analysed by IB. (f) Lysates from HT29 and SW620 cells infected with the indicated viruses were analysed by IB. (g,h) SLAP inhibition potentiates SRC-induced cell transformation and EPHA2 phosphorylation on Tyr. (g) HCT116 cells were infected with the indicated viruses. Cell lysates were IP with an anti-EPHA2 antibody. WCL and immunoprecipitates were analysed by IB. (h) Left panel: soft agar colony formation assay. Right panel: invasion assay. Data represent means±s.e.m.;n=3; **P<0.01, ***P<0.001 (Student’sttest). (i) CRC cells with a low SLAP expression show a higher sensitivity to SRC inhibitors. HCT116 cells that express anti-SLA(shSLAP-2) or anti-Luciferase (shLuc) shRNAs were treated with the SRC inhibitors PP2 (5 μM), PP1 (5 μM), SU6656 (5 μM) or vehicle (DMSO). Left panel: soft agar assays; histograms show the percentage of colonies obtained from indicated cells relative to control cells (treated with DMSO). Right panel: Boyden chamber assays; histograms show the percentage of invasion of indicated cells compared with control (cells treated with DMSO). Data represent means±s.e.m.;n=4. *P<0.05, **P<0.01 (Student’sttest). Figure 8: SLAP controls the SRC oncogenic potential and the cell response to SRC inhibitors. ( a , b ) The interaction between SLAP and EPHA2 is SRC-dependent. ( a ) HEK293T were transfected with the indicated constructs and with siRNA targeting SRC (+) or siRNA negative control (−). 72 h after transfection, cell lysates were immunoprecipitated (IP) with the indicated antibodies. Whole-cell lysates (WCL) and immunoprecipitates were analysed by immunoblotting (IB). ( b ) HT29 cells expressing SLAP or not were treated with the SRC inhibitor PP2 (5 μM) or vehicle (DMSO) for 4 h. Cell lysates were IP with the indicated antibodies. WCL and immunoprecipitates were analysed by IB. ( c ) SRC phosphorylates EPHA2 in vitro . Indicated proteins were incubated with or without ATP. The levels of pY594-EPHA2, EPHA2 and SRC were analysed by IB. ( d – f ) SRC mediates SLAP-dependent EPHA2 destabilization. HT29 cells that express SLAP or not ( d ) and HCT116 cells ( e ) were treated with the SRC inhibitors PP1 (5 μM), PP2 (5 μM) or vehicle (DMSO) for 4 h. Cell lysates were analysed by IB. ( f ) Lysates from HT29 and SW620 cells infected with the indicated viruses were analysed by IB. ( g , h ) SLAP inhibition potentiates SRC-induced cell transformation and EPHA2 phosphorylation on Tyr. ( g ) HCT116 cells were infected with the indicated viruses. Cell lysates were IP with an anti-EPHA2 antibody. WCL and immunoprecipitates were analysed by IB. ( h ) Left panel: soft agar colony formation assay. Right panel: invasion assay. Data represent means±s.e.m. ; n =3; ** P <0.01, *** P <0.001 (Student’s t test). ( i ) CRC cells with a low SLAP expression show a higher sensitivity to SRC inhibitors. HCT116 cells that express anti- SLA (shSLAP-2) or anti-Luciferase (shLuc) shRNAs were treated with the SRC inhibitors PP2 (5 μM), PP1 (5 μM), SU6656 (5 μM) or vehicle (DMSO). Left panel: soft agar assays; histograms show the percentage of colonies obtained from indicated cells relative to control cells (treated with DMSO). Right panel: Boyden chamber assays; histograms show the percentage of invasion of indicated cells compared with control (cells treated with DMSO). Data represent means±s.e.m. ; n =4. * P <0.05, ** P <0.01 (Student’s t test). Full size image SLAP controls the SRC oncogenic potential in CRC cells We next assessed the contribution of this feedback loop to the oncogenic potential of SRC in CRC cells. Remarkably, while SRC catalytic activity was not modified by SLAP expression in HCT116 cells, its oncogenic potential was dramatically enhanced upon SLA silencing ( Fig. 8h ). This biological effect was accompanied by a robust increase in pTyr-EPHA2 level ( Fig. 8g ) and EPHA2 silencing reduced the oncogenic potential of SRC induced by SLAP inactivation ( Supplementary Fig. 12 ), demonstrating that EPHA2 signalling is instrumental to this process. We thus concluded that SLAP defines an additional important mechanism for the control of SRC oncogenic signalling through the destabilization of specific SRC substrates. Our model would therefore predict that cells displaying aberrantly high SRC activity in a context of low SLAP expression should demonstrate a high sensitivity to SRC inhibitors. Indeed, we found that while the SRC inhibitors PP1, PP2 and SU6656 induced a partial reduction of cell-transforming properties of HCT116 cells, this cell response was greatly enhanced in cells where SLA was silenced ( Fig. 8i ). A similarly powerful effect was obtained with the inhibition of the SRC substrate EPHA2 using an RNA interference strategy ( Supplementary Fig. 13 ). Altogether these data are consistent with the notion that SRC inhibitors may be particularly active in patients whose tumours exhibit a high SRC activity together with a low SLAP expression. Our study reveals a novel function of SLAP in human malignancy and shows that SLAP has a tumour-suppressive role in CRC. It also confirms that this adaptor is an important negative regulator of SRC-like signalling. SLAP inactivation primarily involves inhibition of gene expression and in some cases loss-of-function mutations (detected in 2% of CRC) that may inhibit the function of the SH2 and SH3 domains [31] , [32] . Therefore, these mutations may have a significant biological incidence on malignant progression. Our work also uncovered a novel mechanism by which SLAP antagonizes SRC-dependent signalling independently of CBL. By associating with the ubiquitin factor UBE4A, SLAP promotes the destabilization of EPHA2, an important SRC oncogenic substrate in CRC cells ( Fig. 9 ). The relevance of this mechanism in human disease is supported by the inverse correlation observed between SLAP expression level and EPHA2 protein level in human tumour samples and by the capacity of EPHA2 to antagonize SLAP function. This novel mechanism is reminiscent of the way SLAP controls TCR expression by interacting with the E3 ligase CBL [20] and suggests that a major SLAP function may be to promote the destabilization of SFK substrates. UBE4A belongs to the U box-containing protein family and was without a clearly assigned function. Here we show that UBE4A has a tumour suppressor function, possibly through inhibition of a SRC/EPHA2/AKT oncogenic signalling cascade required for malignant transformation. This notion is consistent with previous reports showing that UBE4A gene mutations occur in human cancer [33] and that auto-antibodies against this factor are associated with the severity of Crohn’s disease [34] . A different situation was described for UBE4B, a close relative of UBE4A that promotes HDM2-mediated degradation of the tumour suppressor p53 leading to cell transformation. To our knowledge, UBE4A and EPHA2 are the first proteins to be identified as binding to SLAP SH3. It was previously shown that SLAP SH3 and SH2 are required for attenuating TCR signalling [19] , but the underlying mechanism was not addressed. We hypothesize that UBE4A, through binding to SLAP SH3, could be also an important downstream component of this signalling process. Clearly additional functions for UBE4A may be unravelled in non-transformed cells. 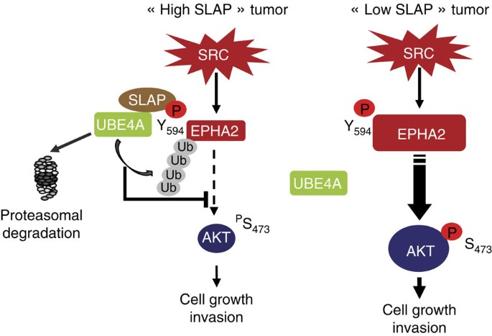Figure 9: A model for SLAP anti-oncogenic activity in the control of SRC oncogenic potential in CRC cells. A model depicting SLAP tumour supressor functions in CRC where SLAP promotes destabilization of specific SRC oncogenic substrates involved in cell tumorigenicity and metastasis. In tumours expressing a high level of SLAP, SRC hyperactivation phosphorylates EPHA2 on Tyr594 that creates a binding site for SLAP SH2 promoting EPHA2/SLAP/UBE4A complex formation and EPHA2 proteasomal degradation. EPHA2 destabilization limits SRC/EPHA2/AKT oncogenic signalling involved in cell tumorigenicity and invasiveness. In tumours expressing low level of SLAP, this negative-feedback loop is inactivated, EPHA2 protein is stabilized and SRC/EPHA2/AKT oncogenic signalling is increased. Therefore, SLAP expression in CRC dictates the oncogenic addiction of tumour cells to a SRC-dependent signalling. Figure 9: A model for SLAP anti-oncogenic activity in the control of SRC oncogenic potential in CRC cells. A model depicting SLAP tumour supressor functions in CRC where SLAP promotes destabilization of specific SRC oncogenic substrates involved in cell tumorigenicity and metastasis. In tumours expressing a high level of SLAP, SRC hyperactivation phosphorylates EPHA2 on Tyr594 that creates a binding site for SLAP SH2 promoting EPHA2/SLAP/UBE4A complex formation and EPHA2 proteasomal degradation. EPHA2 destabilization limits SRC/EPHA2/AKT oncogenic signalling involved in cell tumorigenicity and invasiveness. In tumours expressing low level of SLAP, this negative-feedback loop is inactivated, EPHA2 protein is stabilized and SRC/EPHA2/AKT oncogenic signalling is increased. Therefore, SLAP expression in CRC dictates the oncogenic addiction of tumour cells to a SRC-dependent signalling. Full size image Our report reveals a new mechanism of SRC oncogenic activity in human cancer that involves the inactivation of the adaptor protein SLAP promoting stabilization of a specific SRC substrate. These data bring forward the main concept that deregulation of the catalytic activity of SRC is not sufficient to induce cell transformation but that stabilization of cognate substrates plays an essential additional role in this process. In addition, our data are consistent with a model where SRC oncogenic induction is achieved through inactivation of SRC feedback loops, which may explain, at least in part, why SRC oncogenic mutations are rare in human cancer. In CRC cells, SRC catalytic deregulation is induced by disruption of a SRC feedback loop via silencing of the CSK regulator Cbp/PAG [7] , [8] and we show that stabilization of the SRC oncogenic substrate EPHA2 is also induced by disruption of a SRC regulatory loop through SLA silencing. Consequently, upregulation of wild-type SRC in advanced tumour stages may be sufficient to induce oncogenic signalling. A previous phosphoproteomic analysis revealed that SRC phosphorylates a cluster of TK, including the receptors MET and EPHA2 that mediate CRC cell tumorigenicity and invasiveness [11] . How SRC elicits the activation of these RTK was previously unclear but the present study describes a mechanism that favors SRC–EPHA2 interaction through receptor stabilization following SLAP inactivation. Whether this mechanism also regulates the stability of key additional SRC substrates is an issue that needs to be addressed. Our data also strongly supports the role of EPHA2 as an important downstream component of SRC oncogenic signalling [11] and provides important insight into the mechanism by which EPHA2 promotes ligand-independent oncogenic activity in tumour cells [14] , [35] . EPHA2 malignant signalling can be initiated by AKT-induced phosphorylation on Ser897 (ref. 36 ) or direct interaction with oncogenic RTK by a mostly unknown mechanism [37] , [38] . Here we show that EPHA2 oncogenic function can be induced through its stabilization and phosphorylation on Tyr594 by SRC ( Fig. 9 ). We also reveal that EPHA2 oncogenic signalling in tumour cells is independent from its catalytic activity and from ligand binding. Ligand- as well as some kinase-independent functions of EPHA2 that still required ligand binding have been well documented in cancer cells [39] . In contrast, our data support a novel model where EPHA2 is used by SRC as an adaptor molecule for the recruitment of downstream effectors. In addition, we identified Tyr594 as an important SRC phosphorylation site involved in AKT activation, indicating that in CRC cells, EPHA2 may function as an upstream activator of AKT [14] . Several signalling molecules have been described to associate with this site [40] without any clear link to AKT signalling. We thus anticipate the existence of an additional effector molecule that mediates SRC/EPHA2 signalling, leading to AKT activation. Finally, the finding that EPHA2 is targeted for proteasomal degradation through formation of a SLAP–UBE4A–EPHA2 complex highlights a mechanism that is independent of CBL signalling and Ephrin binding. We thus hypothesize that SLAP targets an EPHA2 pool that is different from the one displaying catalytic activity upon ligand binding. Elucidating how this distinct EPHA2 pool mediates SRC oncogenic signalling in the absence of Ephrins will require further investigation. Finally, our results have significant implications for the design of a SRC-targeting therapy in CRC. While several SRC-like inhibitors have been developed, they have so far failed to generate promising results in CRC probably because of the poor stratification of CRC tumours according to their SRC activity levels [6] , [41] . However, results of the present study now imply that the level of SRC deregulation alone may not be sufficient to assess the contribution of SRC oncogenic signalling in tumour cells. Indeed, the level of SLAP downregulation may be a key additional predictor of SRC inhibitor response. Therefore, a high level of SRC activity together with a low level of SLAP expression may provide a rationale to predict CRC response to SRC inhibitors. Antibodies and reagents Antibodies used in this study (dilution for immunoblotting is indicated): anti-SLAP clone C-19 (sc-1215, 1:500), anti-EPHA2 clone C-20 (sc-924, 1:1,000), anti-FAK pY861 (sc-16663, 1:1,000) anti-UBE4A clone G-20 (sc-54554, 1:500) and anti-CBL clone C-15 (sc-170, 1:1,000) from Santa Cruz Biotechnology; anti-ERK1/2 clone 137F5 (no. 4695, 1:1,000), anti-ERK1/2 pT202/Y204 (no. 4370, 1:1,000), anti-EPHA2 pY594 (no. 3970, 1:1,000), anti-AKT (no. 9272, 1:1,000), anti-AKT pS473 clone D9E (no. 4060, 1:1,000) and anti-pTyr clone pY100 Sepharose bead conjugate (no. 9419) from Cell Signaling Technology; anti-SRC pY418 (no. 44660G, 1:1,000), anti-Ubiquitin clone Ubi-1 (no. 13-1600, 1:1,000) and anti-goat Alexa-594 (no. A11080; 1,000) from Life technologies; anti-FAK (no. 06-543, 1:1,000) from Upstate Biotechnology; anti-pTyr clone 4G10 Agarose conjugate (no. 16-101) from Millipore; anti-Flag (no. F7425, 1:1,000) and anti-Flag M2 Agarose affinity gel (A2220) from Sigma Aldrich; anti-Tubulin (hybridoma gift from N. Morin, CRBM, Montpellier, France, 1:2,000); anti-pTyr 4G10 (hybridoma gift from P. Mangeat, CRBM, Montpellier, France, 1:50); anti-SFK described in ref. 8 (1:1,000); anti-rabbit IgG-HRP (no. NA934, 1:5,000) and anti-mouse IgG-HRP (no. NXA931, 1:5,000) from GE Healthcare; anti-goat IgG-HRP (no. P0449, 1:5,000) from Dako. SU6656 (no. 572636) and Akti-1/2 (no. 124017) were purchased from Calbiochem. PP1 (no. P0040), PP2 (no. P0042), MG132 (no. M7449), E-64 (no. E3132), Leupeptin (no. L2884) Chloroquine (no. C6628), NH4Cl (no. A9434) and Pepstatin A (no. P5318) were from Sigma Aldrich. Recombinant Ephrin-A1-Fc (no. 602-A1-200) was purchased from R&D Systems. Plasmids The pcDNA3-SLAP-Flag, SLAP SH3*(P73L)-Flag, SLAP SH2*(R111E)-Flag and SLAP SH3*SH2*-Flag constructs were obtained from A. Weiss (University of California, San Francisco, USA). The pcDNA3-SLAP N32-Flag and SLAP G2A-Flag constructs encoding SLAP-Flag deleted from aa 161–281 and G to A substitution in the myristylation site of Slap-Flag respectively were described in ref. 42 . SLAP-Flag and its mutants were subcloned in the pMX-pS-CESAR retroviral vector. The pMX-pS-CESAR construct encoding human SRC was previously described [11] . SRC was subcloned in the pBABE retroviral vector. The pcDNA3 construct that expresses mouse EPHA2 (a gift from J. Chen, Vanderbilt University, Nashville, USA), EPHA2 Y594F and EPHA2 Kinase Dead (KD) vectors that were generated by PCR using the QuickChange Site-Directed Mutagenesis Kit (Stratagene) and the following oligonucleotides: 5′-TGTGGATCCTCACACTTTCGAAGACCCCAACC-3′ and 5′-GATACCGGTGGCCATCGCGACACTGAAAGCGGGC-3′, respectively, were subcloned in pBABE. Human UBE4A cDNA was obtained from an ORFeome library and was cloned in pcDNA3. pcDNA3 encoding UBE4A PA mutant, which corresponds to the inactive form of the ligase due to the replacement of Pro1030 into Ala, was obtained by PCR using the QuickChange Site-Directed Mutagenesis Kit (Stratagene) and the following oligonucleotide: 5′-TGCTCAGTGACCAAACAGATGCCTTTAACCGTAGT-3′. SLAP N32 and SLAP N3*2 were subcloned in the pGEX vector. The GST-UBE4A construct was obtained from K.-I. Nakayama (Medical Institute of Bioregulation, Kyushu University, Fukuoka, Japan) and pRBG4 Ubiquitin-myc-6His from J. Pierre (IGR, Université Paris-XI, France). The shRNA sequences used are listed in Supplementary Table 2 and were cloned in the pSiren-retroQ or pRETRO-SUPER.neo.GFP retroviral vector according to the manufacturer’s instructions (Clontech). Constructs expressing a scramble shRNA (shmock) or a shRNA directed against Luciferase (shLuc) were used as negative controls. Human tissue collection Specimens of colon tumours (17 patients) and histologically normal epithelium were obtained from the pathologist after resection according to the French government regulations and with the approval by the relevant Ethics Committee (CHU Carémeau, Nîmes, France). Informed consent was obtained from all patients. Tissue samples were stored in liquid nitrogen until further use. Tissue sections were prepared from liquid nitrogen-frozen tumour samples as described in ref. 43 . Briefly, laser capture microdissection was performed using a PixCell IIe microdissector (Arcturus/Alphelys, Plaisir, France) with the following settings: 265 mV, 45 mWh, 15 μm diameter, 1.8 ms. RNA was prepared from microdissected tissues using the RNAeasy Microkit (Qiagen). The quality and amount of RNA recovered were assessed using RNA pico Labchips (Agilent Technologies). Protein extraction from frozen tissues was performed at 4 °C in lysis buffer using a Duall Glass Tissue Grinder size 21. Cell culture and transfections All cell lines were obtained from the American Type Culture Collection (ATCC, Rockville, MD, USA) and were cultured at 37 °C and 5% CO 2 in a humidified incubator in specific growth medium (Invitrogen) supplemented with 10% fetal calf serum (FCS), 100 U ml −1 penicillin and 100 μg ml −1 streptomycin. The culture media used were: RPMI 1640 Medium Glutamax for Jurkat, Colo205 and LS174T cells; Dulbecco’s Modified Eagle’s Medium (DMEM) Glutamax for CoN CCD 841, IMR-90, HT29, HCT116, SW480, SW620, Lovo, Co115, DLD1, HEK293T and NIH3T3 cells; DMEM-F12 Glutamax for T84 cells. Retroviral infections Retroviral infections were described in ref. 8 and stable cell lines were obtained in a polyclonal background by selection with 1 μg ml −1 puromycin or 800 μg ml −1 geneticin or by fluorescence-activated cell sorting. Transient plasmid transfections in HEK293T cells were performed with the jetPEI reagent (Polyplus-transfection) according to the manufacturer’s instructions. siRNAs (Dharmacon) were transfected with the Lipofectamine 2000 reagent (Invitrogen) (HEK293T and NIH3T3 cells) or with JetPEI (Polyplus-transfection) (HT29 and SW620 cells). For transfection with Lipofectamine 2000, 10 6 cells were seeded in 60-mm dishes and transfected according to manufacturer’s protocol using 300 pmol siRNA and 8 μl Lipofectamine. For transfection with JetPEI, 15 × 10 4 cells were seeded in six-well plates and transfected according to manufacturer’s protocol using 150 pmol siRNA and 8 μl JetPEI. The siRNA sequences used are listed in Supplementary Table 2 . A scramble siRNA (simock) or a siRNA directed against Luciferase (siLuc) were used as negative controls. RNA extraction and quantitative RT–PCR mRNA was extracted from cell lines and tissue samples using the TRIzol reagent (Invitrogen), including DNase treatment (Qiagen), according to the manufacturer’s instructions. RNA (1 μg) was reverse transcribed with MMLV reverse transcriptase (Invitrogen). qPCR was performed with the SyBR Green Master Mix in a LightCycler 480 (Roche). The expression levels were normalized to mouse Gapdh and ActinB expression and to human GAPDH and B2M expression and analysed using the ΔΔ C t method. Primers used for qPCR are listed in Supplementary Table 3 . Immunofluorescence staining Paraffin-embedded sections were deparaffinized and rehydrated. Antigens were retrieved by boiling sections in 10 mM citrate buffer (pH 6.0) for 20 min. Sections were blocked with 5% milk in PBS containing 0.5% Triton X-100 and were incubated at 4 °C with anti-SLAP antibody (1:50) overnight followed by anti-goat Alexa-594 (1:500) at room temperature for 1 h. Images were taken using a Leica DM6000 microscope with a Leica × 10 HC PL APO 0.4 CS objective. Biochemistry Immunoprecipitation (IP) and immunoblotting (IB) were performed as described [8] . Briefly, cells were lysed at 4 °C with lysis buffer (20 mM Hepes (pH 7.5), 150 mM NaCl, 0.5% Triton X-100, 6 mM β-octylglucoside, 10 μg ml −1 aprotinin, 20 μM leupeptin, 1 mM NaF, 1 mM DTT and 100 μM sodium orthovanadate). IP was performed with 500 μg proteins and 2 μg of the specific antibody. Immunoprecipitates or 20–50 μg of whole-cell lysates were loaded on SDS–PAGE gels and transferred onto Immobilon membranes (Millipore). Detection was performed using the ECL System (Amersham Biosciences). Larger images of all immunoblots shown in the main article are included in Supplementary Fig. 14 . Band intensity was quantified by the ImageJ software, protein levels were normalized to control and quantifications are shown in Supplementary Fig. 15 . For GST pull-down assays, the expression of fusion proteins in Escherichia coli (BL21 strain) was induced by incubation with 0.2 mM isopropyl β- D -thiogalactopyranoside (IPTG) at 25 °C for 3 h (GST-SLAP N32 and GST-SLAP N3*2) or at 16 °C overnight (GST-UBE4A). The expressed proteins were purified as described in ref. 44 and bound to Glutathione Sepharose 4B beads (GE Healthcare). GST fused to UBE4A was cleaved using the PreScission Protease according to the manufacturer’s instructions (GE Healthcare). Fifteen micrograms of GST alone, GST-SLAP N32 and GST-SLAP N3*2 bound to Glutathione Sepharose beads were incubated with 5 μg of UBE4A at 4 °C for 2 h. Complexes were washed in PBS and analysed by IB. For ubiquitination assays in cellulo , HEK293T cells were lysed at room temperature with urea buffer (20 mM Tris–HCl (pH 7.5), 200 mM NaCl, 10 mM Imidazole, 0.1% Triton X-100 and 8 M urea). Ubiquitinated proteins were purified using cobalt beads (Clontech). Complexes were washed in urea buffer and then PBS and analysed by IB. For ubiquitination assays in vitro , 20 μg of Ubiquitin (Sigma Aldrich), 0.1 μg of E1 produced in baculovirus, 1 μg of UbcH5B produced in bacteria, 83.5 ng of UBE4A-Flag (Origen Technologies), 15 ng of SLAP N32 produced in bacteria, 50 ng of EPHA2 cyto -GST (cytoplasmic domain: aa 560–976 of EPHA2 fused to GST, Invitrogen), 20 mM Tris–HCl (pH 7.5), 5 mM MgCl 2 , 1 mM ATP and 1 mM dithiothreitol were incubated for 1 h at 37 °C. The reaction was terminated by the addition of SDS sample buffer containing β-mercaptoethanol and heating at 95 °C for 5 min. Kinase assays were perform using 200 ng of purified EPHA2 recombinant protein (OriGen Technologies), in the absence or presence of 50 ng of the purified kinase domain of SRC (a generous gift from G. Labesse, CBS, Montpellier, France) and in the absence or presence of 0.1 mM ATP Lithium Salt (Roche Diagnostics) in kinase buffer (20 mM Hepes (pH 6.5), 10 mM MnCl 2 , 1 mM DTT) for 10 min at 30 °C. SILAC-based quantitative proteomic SW620 cells were cultured in SILAC DMEM (Pierce) without Lysine (Lys) and Arginine (Arg) and supplemented with 4 mM L -glutamine, 10% dialyzed FBS (Invitrogen), 0.084 g l −1 Arg and 0.146 g l −1 Lys. Heavy ( 13 C 6 15 N 4 -Arg and 13 C 6 15 N 2 -Lys, from EurisoTop) or unlabelled amino acids (light Arg and Lys, from Sigma Aldrich) were used. After 3 weeks of metabolic labelling, cells were lysed in lysis buffer. Heavy and light lysates (30 mg of protein) were mixed and immunoprecipitated with anti-Flag M2 agarose overnight at 4 °C. IP were eluted using 500 μg ml −1 Flag peptide (in TBS) for 30 min 4 times. pTyr proteins were immunoprecipitated with a mixture of the 4G10 and pY100 antibodies overnight at 4 °C. Proteins from single or double purifications were separated by SDS–PAGE and trypsin-digested samples (1 μl) obtained from nine cut gel slices were analysed by LC-MS/MS on a LTQ-Orbitrap mass spectrometer (ThermoFisher) as previously described [11] . Briefly, peptides were analysed online by nano-flow HPLC (U3000, Dionex) nanoelectrospray ionization. Desalting and pre-concentration of samples were performed online on a Pepmap pre-column (0.3 mm × 10 mm, Dionex). A gradient consisting of 0–40% B in A for 60 min, followed by 80% B/20% A for 15 min (A=0.1% formic acid, 2% acetonitrile in water; B=0.1% formic acid in acetonitrile) at 300 nl min −1 was used to elute peptides from the capillary reverse-phase column (0.075 × 150 mm, Pepmap, Dionex). All MS/MS spectra were recorded using normalized collision energy (35%, activation Q 0.25 and activation time 10 ms) with an isolation window of 2 m / z . Raw data analysis was performed using the MaxQuant software (v. 1.1.1.14) using standard settings and the SwissProt_Human database (release 2010_10; http://www.uniprot.org , 20,259 entries), 255 frequently observed contaminants as well as reversed sequences of all entries. Soft agar colony formation assay A total of 1,000 cells per well were seeded in 12-well plates in 1 ml DMEM containing 10% FCS and 0.33% agar on a layer of 1 ml of the same medium containing 0.7% agar. Cells were treated with vehicle alone or the indicated drugs every 3 days. After 18–21 days, colonies with >50 cells were scored as positive. Invasion assay Cell invasion assays were performed in Boyden chambers (BD Bioscience) using 60,000 cells in the presence of 100 μl Matrigel (0.33 mg ml −1 ; BD Bioscience). After 48 h, cells were fixed in 3.7% paraformaldehyde solution containing 0.1% Hoechst. Whole-well images were acquired using an inverted microscope (Zeiss Axiovert 200 M or Leica DMIRE2) and a × 10 EC Plan Neofluar 0.3 PH1 objective. Nuclei were then counted in whole wells using the Metamorph software (Molecular Devices, Inc.). In vivo experiments In vivo experiments were performed in compliance with the French guidelines for experimental animal studies (Direction des Services Vétérinaires, Ministère de l’Agriculture, Agreement no. B 34-172-27) and fulfilled the UK Coordinating Committee on Cancer Research guidelines for the welfare of animals in experimental neoplasia. For the subcutaneous xenograft model: 2 × 10 6 cells were injected into the flank of 6–7 week/old female Swiss nu/nu ( nude ) mice (Charles River). After 35 days, tumours were excised, weighed and cryopreserved. For the liver metastasis model: 1.5 × 10 6 cells were injected in the spleen of 5–6-week/old female BALB/c nu/nu mice (Charles River). Two minutes after injection, the spleen was removed to prevent the formation of primary tumours. After 3 weeks, the liver was removed, photographed and cryopreserved. For siRNA experiments: APC Δ14/+ mice were a generous gift from C. Perret (Institut Cochin, Paris, France). Before use, siRNAs were complexed with cationic liposomes (a generous gift from V. Escriou, Paris Descartes University, France) [45] : equal volumes of cationic liposomes (60 nmol) and siRNA (10 μg) in 0.9% NaCl were mixed and incubated at room temperature for 30 min. Then, 3-week old APC Δ14/+ mice received i.p. injections of siRNA twice a week for 6 weeks. Five days after the last injection, intestinal tumours were counted, measured, removed and cryopreserved. Statistical analysis All analyses were performed using GraphPad Prism. Data are presented as the mean±s.e.m. When distribution was normal (assessed with a Shapiro–Wilk test), the two-tailed t -test was used for between group comparisons. In the other cases, the Mann–Whitney test was used. The Pearson coefficient was calculated to determine the correlation between the normally distributed SLAP mRNA and EPHA2 protein expressions in human tumours. Statistics were carried out on a minimum of three independent experiments. The statistical significance level is illustrated with P -values: * P ⩽ 0.5, ** P ⩽ 0.01 and *** P ⩽ 0.001. How to cite this article: Naudin, C. et al . SLAP displays tumour suppressor functions in colorectal cancer via destabilization of the SRC substrate EPHA2. Nat. Commun. 5:3159 doi: 10.1038/ncomms4159 (2014). Accession codes: The proteomics data have been deposited in the peptide atlas under the accession code PASS00376.